Nanophotonic integrated circuits from nanoresonators grown on silicon Harnessing light with photonic circuits promises to catalyse powerful new technologies much like electronic circuits have in the past. Analogous to Moore’s law, complexity and functionality of photonic integrated circuits depend on device size and performance scale. Semiconductor nanostructures offer an attractive approach to miniaturize photonics. However, shrinking photonics has come at great cost to performance, and assembling such devices into functional photonic circuits has remained an unfulfilled feat. Here we demonstrate an on-chip optical link constructed from InGaAs nanoresonators grown directly on a silicon substrate. Using nanoresonators, we show a complete toolkit of circuit elements including light emitters, photodetectors and a photovoltaic power supply. Devices operate with gigahertz bandwidths while consuming subpicojoule energy per bit, vastly eclipsing performance of prior nanostructure-based optoelectronics. Additionally, electrically driven stimulated emission from an as-grown nanostructure is presented for the first time. These results reveal a roadmap towards future ultradense nanophotonic integrated circuits. Densely integrating devices on a single chip enables both complex functionality and economy of scale. This principle has been a driving force for the electronics industry [1] , and it is certain to translate to photonic integrated circuits (PICs) as well [2] . By combining components that generate, detect and otherwise control light, PICs facilitate design of photonic architectures that prove far more powerful than any single photonic element alone. Already, they have sparked great interest for communications and computing technology [3] , [4] . Other rapidly emerging applications meanwhile include light detection and ranging [5] , optofluidics [6] and more. Though semiconductor fabrication technology has empowered silicon electronics to scale, nanostructure growth perhaps provides a more viable approach for photonics [7] . Active photonic devices rely heavily on III–V materials because of their proficiency for controlling optical processes [8] , yet etching small III–V structures debilitates material quality because of III–V compounds’ sensitivity to surface conditions [9] . While SiO 2 offers remarkable surface passivation properties for silicon [10] , a comparable solution for III–V semiconductors remains absent. On the other hand, low-defect single-crystal nanostructures can be grown with atomically flat surfaces and in situ surface passivation via higher band gap cladding layers [11] , [12] , which have historically proven to provide the best passivation for III–V materials. With tiny footprints, nanostructures incur minimal real estate cost while offering full photonic functionality. Furthermore, optoelectronic devices in PICs require a diverse set of materials, and nanostructure growth has proven promising for heterogeneous material integration [13] , [14] . Nonetheless, shrinking photonics has thus far demanded major tradeoffs in performance and practicality. In particular, though a wide range of optical operations have been achieved with nanowires, most experiments required optical control [15] , [16] , [17] . Meanwhile, PIC applications will likely necessitate electrically controllable optoelectronic devices. A few demonstrations of nanowire optoelectronics exist, but either single nanowires were removed from their native substrates [18] , [19] , [20] or nanowire ensembles were used [21] , [22] . Both scenarios make mass device integration extremely demanding. Thus, it is no wonder that using such devices in circuit- and system-level experiments has been out of reach. Ironically, a driving factor behind relatively poor past performance from nanowires is that they are perhaps simply too small. Conventional nanowires are limited to critical diameters [23] of only 10–200 nm in width. Robustness and precision consequently become issues during harsh fabrication processes used to electrically contact monolithic single nanowires. Highly subwavelength dimensions also result in poor optical confinement, inhibiting optoelectronic device performance, particularly around making lasers and high-responsivity photodetectors. If similar structures can be created with wavelength-scale dimensions, many of these challenges can be mitigated. Recently, we showed that this is possible via growth of InGaAs nanopillars on silicon. Though they first nucleate as nanoneedles only a few nanometres wide [24] , [25] , they can scale well beyond 1 μm in diameter while remaining single crystalline [13] , [26] . Exhibiting strong optical cavity effects, these structures are natural nanoresonators [27] . In this article, these nanoresonators provide a platform for all primary optoelectronic functions as embodied by an I – V characteristic’s three operational quadrants: light emission (+ I , + V ), light detection (− I , − V ) and energy generation (− I , + V ). We demonstrate nanoresonator device performance within the realm of state-of-the-art numbers, validating nanostructures as a promising approach to scaling down dimensions of future photonic devices. Finally, as schematized in Fig. 1a , we construct functional optical links on a silicon substrate from nanoresonators to explore applications to photonic circuits for the first time. 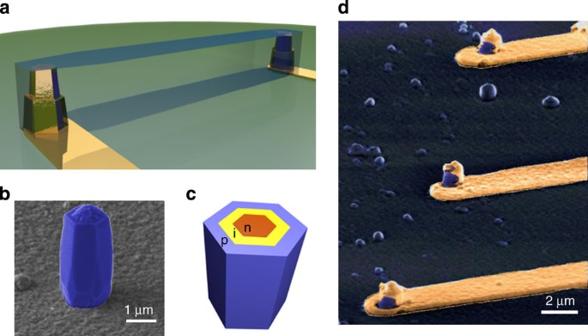Figure 1: Assembling photonic circuits via nanostructure growth. (a) A schematic of an optical link formed by interconnecting two optoelectronic devices fabricated from GaAs-based nanoresonator structures grown on silicon. (b) An SEM image shows the hexagonal nature of the as-grown resonator. (c) Through core-shell growth, radial p–i–n junctions form within each structure, providing the basis of our nano-optoelectronic devices. (d) An SEM image shows a fabricated array of such devices. Figure 1: Assembling photonic circuits via nanostructure growth. ( a ) A schematic of an optical link formed by interconnecting two optoelectronic devices fabricated from GaAs-based nanoresonator structures grown on silicon. ( b ) An SEM image shows the hexagonal nature of the as-grown resonator. ( c ) Through core-shell growth, radial p–i–n junctions form within each structure, providing the basis of our nano-optoelectronic devices. ( d ) An SEM image shows a fabricated array of such devices. Full size image Nanoresonators directly grown on silicon Growth of nanoresonators on silicon occurs via metal-organic chemical vapour deposition (MOCVD) at a low temperature of 400 °C without metal catalysts. Notably, these conditions are favourable for CMOS devices, raising the possibility of integrating III–V PICs with silicon electronics. Additional details on the nanomaterial synthesis process can be found in both references [24] , [27] and the Methods section. Figure 1b displays a scanning electron microscope (SEM) image of a single as-grown InGaAs nanoresonator, showcasing the hexagonal nanopillar geometry that provides a natural optical cavity. A key development enabling the high-performance devices presented in this article lies in the improved diode junctions grown inside nanoresonators. Already, ideality factors approach 2 for this nascent nanomaterial ( Supplementary Fig. 1 and Supplementary Note 1 ). As suggested in the cross-section schematic of Fig. 1c , radial heterojunctions are created by varying doping and composition during core-shell growth. Typically, the diode structure consists of an n-doped In 0.12 Ga 0.88 As core, a 20–30% indium intrinsic In x Ga 1− x As active layer, and a p-doped GaAs outer shell providing both electrical contact and surface passivation. In addition, we note that the doping concentration exhibits excellent uniformity along the axial direction due to the characteristic core-shell growth mechanism, as illustrated by Supplementary Figs 2 and 3 . More discussions can be found in Supplementary Note 2 . Armed with these diode junctions, individual nanoresonators can each form a single optoelectronic device. Their robustness and form factor meanwhile make them highly compatible with traditional nanofabrication processes, which are used to electrically contact these structures. Figure 1d shows an SEM image of several nanoresonator optoelectronic devices. Additional details on both the diode structure and device fabrication can be found in the Methods section. Electrically driven stimulated emission Light emitters are paramount for generating photons that propagate through optical circuits and media. Under optical pumping, our nanoresonator structures lase due to strong resonances supported by their natural geometry [27] . However, PICs require optoelectronic devices with electrical control, and electrical contacts greatly perturb these cavity modes, making electrically driven lasing a difficult task. By embedding our nanoresonator structure inside a metal-optic cavity [28] , [29] , [30] , we show that nanoresonator produces electrically driven stimulated emission. Although stimulated emission is observed under both continuous wave (CW) and pulsed pumping, full laser oscillation has not yet been achieved. However, achieving electrically driven stimulated emission represents a great milestone and monumental leap towards realizing electrically injected nanolaser on silicon. In an integration scheme as depicted in Fig. 2a , we fabricated metal contact on the nanoresonator that doubles as both an electrical contact and a metal mirror. 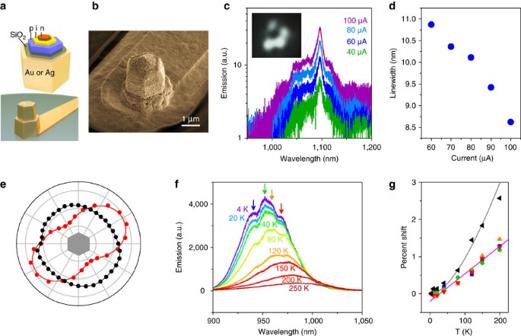Figure 2: Stimulated emission from resonant LEDs. (a) A schematic illustrates how as-grown nanoresonators can be embedded in metal-optic cavities as a step towards electrically driven nanolasers on silicon. (b) An SEM image shows a fabricated LED with a gold metal-optic cavity. (c) Devices exhibit stimulated emission peaks in their spectra under progressively higher CW injection levels at 4 K. The inset shows an image of stimulated emission, revealing an apparent mode pattern. This particular device used silver encapsulation and a nominal 30% indium active layer. (d) Linewidth of the stimulated emission peak as a function of injection current. The linewidth is calculated by fitting the emission spectra in (c) with a Gaussian function representing the spontaneous emission, and a Lorentzian function representing the stimulated emission peak. (e) While photoluminescence from as-grown nanopillars (black) shows no obvious polarization dependence, the spectral peak near 1.1 μm in (c) is highly polarized (red), further ascribing its origin to cavity mode amplification. The hexagon in the centre indicates the nanopillar crystal orientation relative to the polarization angle measured. (f) Temperature dependence experiments shed insight into the origin of peaks, highlighted by the coloured arrows, in device spectra. The spectra incandfare from two different devices. Panelgexplicitly shows how the peaks redshift versus temperature. Coloured symbols correspond to peaks labelled by similarly coloured arrows inf. The peaks shift at the same rate expected for refractive index of InGaAs (dn/dT=2.67 × 10−4) as plotted by the pink line. This confirms that the peaks are due to cavity resonances, which depend linearly on refractive index. Meanwhile, the temperature dependence of the overall background spontaneous emission (black triangles) follows the well-known Varshni model for energy gaps (plotted as a grey line usingα=4 × 10−4,β=226). Pulsed (20 ns) pumping was used to minimize heating effects in these particular experiments on a gold-encapsulated device with a 20% indium active layer. Figure 2b shows an SEM image of a fabricated device using a gold metal-optic cavity. Gold was initially used as a mirror since it does not oxidize and naturally provides good electrical contact to GaAs-based materials. We later moved onto using silver encapsulation, the metal of choice for metal-optic cavities because of its lower metal loss. Indeed, silver-based devices usually show better performance, though it was beyond the scope of the present work to optimize cavity loss. Stimulated emission has been achieved at 4 K as shown in Fig. 2c . Under progressively higher current injection, a prominent emission peak at ~\n1.1 μm emerges and grows before eventually saturating. Additional cavity modes at shorter wavelengths meanwhile begin to emerge as carrier density builds up inside the nanopillar, thereby increasing and blueshifting material gain. Details on how the emission was recorded can be found in the Methods section. When fitting the emission spectra with a Gaussian function representing the background spontaneous emission and a Lorentzian function representing the cavity peak, the linewidth of the cavity peak is found to narrow from 10.9 to 8.6 nm ( Fig. 2d ). In the inset of Fig. 2c , a top-view image of stimulated emission from a device shows spatial maxima and minima resembling mode patterns, which further suggests that certain modes are indeed amplified and dominate emission. The dark spot in the centre of the image is due to metal inhibiting surface normal light emission. Figure 2: Stimulated emission from resonant LEDs. ( a ) A schematic illustrates how as-grown nanoresonators can be embedded in metal-optic cavities as a step towards electrically driven nanolasers on silicon. ( b ) An SEM image shows a fabricated LED with a gold metal-optic cavity. ( c ) Devices exhibit stimulated emission peaks in their spectra under progressively higher CW injection levels at 4 K. The inset shows an image of stimulated emission, revealing an apparent mode pattern. This particular device used silver encapsulation and a nominal 30% indium active layer. ( d ) Linewidth of the stimulated emission peak as a function of injection current. The linewidth is calculated by fitting the emission spectra in ( c ) with a Gaussian function representing the spontaneous emission, and a Lorentzian function representing the stimulated emission peak. ( e ) While photoluminescence from as-grown nanopillars (black) shows no obvious polarization dependence, the spectral peak near 1.1 μm in ( c ) is highly polarized (red), further ascribing its origin to cavity mode amplification. The hexagon in the centre indicates the nanopillar crystal orientation relative to the polarization angle measured. ( f ) Temperature dependence experiments shed insight into the origin of peaks, highlighted by the coloured arrows, in device spectra. The spectra in c and f are from two different devices. Panel g explicitly shows how the peaks redshift versus temperature. Coloured symbols correspond to peaks labelled by similarly coloured arrows in f . The peaks shift at the same rate expected for refractive index of InGaAs (d n /d T =2.67 × 10 −4 ) as plotted by the pink line. This confirms that the peaks are due to cavity resonances, which depend linearly on refractive index. Meanwhile, the temperature dependence of the overall background spontaneous emission (black triangles) follows the well-known Varshni model for energy gaps (plotted as a grey line using α =4 × 10 −4 , β =226). Pulsed (20 ns) pumping was used to minimize heating effects in these particular experiments on a gold-encapsulated device with a 20% indium active layer. Full size image To better understand the origin of peaks observed in device spectra, we explored their polarization and temperature dependence. As shown in Fig. 2e , the emission peak is polarized as well, which is a signature of stimulated emission and cavity effects. In contrast, basic photoluminescence from as-grown nanopillars exhibits little polarization dependence. Generally, our devices’ resonances tend to be linearly polarized, which may be a by-product of fabrication imperfections perturbing rotational symmetry. To explore the temperature dependence, we turned to another device that shows prominent spontaneous emission with multiple stimulated emission peaks. Figure 2f shows that both the overall spectrum and its superimposed peaks, highlighted by the coloured arrows, redshift versus temperature as might be expected. However, the purported cavity peaks shift at a far slower rate than the spontaneous emission background as elucidated in Fig. 2g . This can be explained by the generally stronger temperature dependence of band gap energy versus that of refractive index. By plotting all wavelength shifts as percentages, we can compare our results to existing models for both types of temperature-dependent phenomena. We see that the redshift of the overall emission spectrum follows the well-known Varshni model using fitting parameter values ( α =4 × 10 −4 , β =226) typical for InGaAs [31] . Meanwhile, the subpeaks redshift at a slower rate that corresponds well to a thermo-optic coefficient of d n /d T =2.67 × 10 −4 , an oft-cited value for GaAs-based materials [32] . Since resonant wavelengths depend linearly on refractive index, this analysis supports that stimulated emission from cavity modes are responsible for the peaks observed in spectra. Though stimulated emission is observed, the nanoresonator device is shy of reaching lasing threshold. Optimizing the metal-optic cavity likely represents the primary roadblock for realizing electrically injected monolithic nanolasers on silicon. Analysis ( Supplementary Fig. 4 ) indicates that material gain as high as 3,400 cm −1 has been demonstrated with current-injected nanoresonators. This implies that quality factors must exceed ~\n100 for lasing, which is trivial for traditional laser structures, but a challenge for nanophotonic cavities. With improved cavity design, an exciting possibility emerges for directly interconnecting nanolasers with PICs and even silicon CMOS circuits. Avalanche photodetectors Optoelectronic applications largely necessitate bidirectional optical–electrical–optical conversion. The inverse process of turning light into electrical signals is therefore just as important as light generation. As shown by the schematic in Fig. 3a and SEM image in Fig. 3b , individual InGaAs nanoresonators can also function as photodetectors. Whereas our previous publication featured ensemble detectors with ~\n30–50 nanoneedles [22] , our current detector uses only a single nanoresonator. This dramatically reduces device footprints from 40,000 to ~\n1 μm 2 , paving the way towards ultra-dense photonic integration. 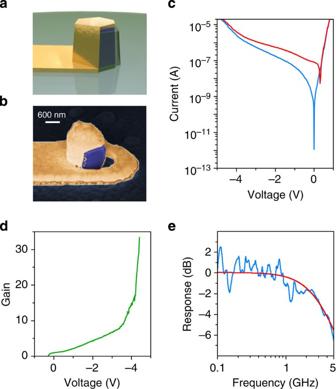Figure 3: Avalanche photodetectors. (a) Schematic of a nanoresonator-based APD. (b) SEM image of a fabricated device. (c)I–Vcurves from a device with (red) and without (blue) incident illumination clearly reveal photocurrent. (d) Strong avalanche gain is observed with increasing reverse bias. At −4.4 V, a multiplication factor of 33 is reached. (e) S21measurements show that the same device with a gain of 33 in (d) has a bandwidth of 3.1 GHz and thereby features a gain-bandwidth product of 102 GHz. Figure 3c shows the I – V curve of a device with dark current of only 1.2 pA at 0 V and 45 nA at −1 V. Some devices exhibit dark current as low as 1 nA at −4 V reverse bias, and many show ideality factors of ~\n2 ( Supplementary Fig. 1 ). Such promising diode performance suggests that III–V nanomaterial quality can approach that of epitaxial films with further development. Under illumination, the I – V curve shifts upwards as seen from the red trace in Fig. 3c , clearly indicating photocurrent generation. Figure 3d shows that photocurrent increases with reverse bias, revealing avalanche multiplication effects. Based on a unity gain current defined by the flat photovoltaic (PV) region near 0 V, avalanche photodetector (APD) gain reaches as high as 33 at −4.4 V. At higher voltages, the APD breaks down and requires proper circuitry to function in Geiger mode. For this particular device, responsivity without gain is modest at only 0.22 A W −1 , though it reaches 7.3 A W −1 at −4.4 V. Improving quantum efficiency of the material will likely improve responsivity in the future, and some devices already show unity gain responsivity as high as 0.6 A W −1 . In our experiments, the wavelength of light (850 nm) limits responsivity to a maximum of 0.68 A W −1 . Thus, with further material development and long wavelength operation, unity gain responsivity approaching 1 A W −1 is entirely possible. Figure 3: Avalanche photodetectors. ( a ) Schematic of a nanoresonator-based APD. ( b ) SEM image of a fabricated device. ( c ) I–V curves from a device with (red) and without (blue) incident illumination clearly reveal photocurrent. ( d ) Strong avalanche gain is observed with increasing reverse bias. At −4.4 V, a multiplication factor of 33 is reached. ( e ) S 21 measurements show that the same device with a gain of 33 in ( d ) has a bandwidth of 3.1 GHz and thereby features a gain-bandwidth product of 102 GHz. Full size image Notably, avalanching occurs at relatively low voltages compared with traditional planar III–V devices. A couple of factors may explain this phenomenon. First, low bias voltages can create very large electric fields given sufficient doping and a small junction width, and our p–i–n junction’s intrinsic region is typically only 200 nm thick. Second, junction curvature effects [33] can enhance the electric field in our radial p–i–n junctions. In our case, we find that low-bias avalanching is more likely due to a thin depletion region rather than junction curvature. Nonetheless, growing radial heterojunctions offers some interesting advantages. Most notably, it effectively allows large area planar diode junctions to be rolled up and planted onto substrates with tiny footprints. The ratio of junction to footprint area is ~\n2 h / r , where h and r are the height and radius of the nanopillar, respectively. Interestingly, this suggests that high aspect ratio nanostructures like the ones presented here can perhaps drive semiconductor device fabrication in a third dimension: upwards [14] . For APDs, a tradeoff exists between gain and bandwidth, thereby making gain-bandwidth product a highly appropriate figure of merit. Here we demonstrate, for the first time, high-speed operation of low-bias voltage nanoresonator APDs [22] . Figure 3e shows a smoothed S 21 response curve for the same device whose multiplication data is displayed in Fig. 3d . The 3-dB bandwidth f 3dB for this device is 3.1 GHz at all bias levels, meaning a 102 GHz gain-bandwidth product is achieved at −4.4 V. S 21 bandwidth is likely independent of bias voltage because device impulse responses feature persistent diffusion tails as shown in Supplementary Fig. 5 . Rise times as fast as 35 ps have been measured for some devices, suggesting 10 GHz bandwidth is possible. However, we have only measured S 21 bandwidths up to 3.8 GHz thus far. In the future, proper optimization of the junction and its characteristics should close this gap by greatly reducing diffusion effects [34] . Additionally, we have thus far neglected the possibility of parasitic elements in the electrical contacts and experimental setup that may further hamper device bandwidth. By addressing these issues, it is well within reason that 300 GHz gain-bandwidth products are possible, finally putting a nanostructure’s performance on par with state-of-the-art bulk devices [35] , [36] . On-chip optical link Photonic circuits require not only components such as emitters and detectors but also a means to interconnect these devices such that they can interact as part of a larger system. Here we have fulfilled this task by converging top–down fabrication technology with our nanoresonator devices. Using electron beam (e-beam) lithography and negative tone resist, we wrote polymer waveguides that coupled a light-emitting diode (LED) on one end to a photodetector on the other. Waveguide lengths were varied but kept short to minimize propagation loss. Since the waveguides themselves were not the core results, we did not optimize their properties for these experiments. 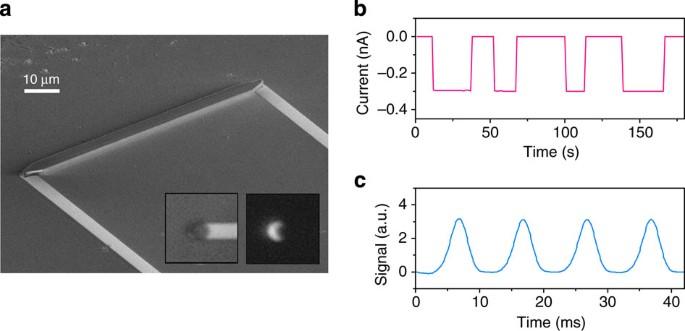Figure 4: Integrated nanophotonic link. (a) SEM image of a nanophotonic link on silicon constructed from nanoresonator devices. The insets show top-view optical images of a single nanoresonator LED and its emission. The optical links clearly and robustly transmit data under both (b) dc operation and (c) ac operation. All link measurements were performed at room temperature. Figure 4a presents an SEM image of the fabricated link, while the insets show optical images of a nanopillar-based LED and its room temperature emission. For optical links, LEDs were metallized on only one side to enable waveguide coupling, contrary to the stimulated emission devices in Fig. 2 . The crescent shape of the light output is due to the one-sided metallization. Figure 4: Integrated nanophotonic link. ( a ) SEM image of a nanophotonic link on silicon constructed from nanoresonator devices. The insets show top-view optical images of a single nanoresonator LED and its emission. The optical links clearly and robustly transmit data under both ( b ) dc operation and ( c ) ac operation. All link measurements were performed at room temperature. Full size image The photonic links were operated under both dc and ac conditions. For the dc experiments, photocurrent can be clearly seen as the LED is turned on and off as shown in Fig. 4b . Approximately 300 pA is generated by the photodetector when the link is turned on, which offers a clear signal, but is a drastic drop from the 400 μA needed to bias the LED. However, minimal effort went into design and optimization of the waveguide for this proof of concept, and thus losses due to waveguide coupling and propagation were likely to be extremely high. For applications involving data transmission or otherwise using pulses of light, photonic links must be able to support ac signals. In Fig. 4e , a 100-Hz optical pulse train is unambiguously delivered from the LED through the waveguide to the photodetector. While 100 Hz is a modest rate, this optical link construction is the first of its kind and holds promise for very densely packing bit streams onto a single chip. Setting aside the space occupied by waveguides, our optical link requires over an order of magnitude less area versus traditional PIC links. The footprints of our emitter and detector together total <10 μm 2 , whereas traditional optoelectronic devices used in PICs need >200 μm 2 at the minimum [37] , [38] . This massive reduction in real-estate cost highlights the possibility of scaling size reduction in future PICs via nanostructure growth. Furthermore, operation at 100 Hz is far from the existing limit of the link. As discussed next, both emitters and photodetectors operate well into the gigahertz regime. Only equipment limitations inhibit higher frequency links from being measured. RF coupling noise between adjacent probes used to bias both ends of the link drown out the photocurrent signal at 1 kHz and beyond. Ultrafast device operation For applications requiring data transmission, particularly in communications and computing, bandwidth and data rates are important measures of performance. In order to test the bandwidth limits of our photonic link, we characterized the dynamics of its component devices. When directly modulated, LEDs can operate at 2.5 Gbit s −1 ( Fig. 5a ). The top trace represents an LED’s response to the bit pattern 10001000. A falling tail can be seen, which likely limits the ultimate bandwidth of the device. The middle trace meanwhile shows the LED emitting an on–off bit pattern, and the bottom curve shows a more diverse pattern of 11001000. The LED successfully reproduced all of the various bit patterns, though greater amplitude variation exists in the last case. On average, the tested device consumed 0.5 mW of power, a low-energy operation of only 0.2 pJ bit −1 . While factors such as link budget certainly must be considered, this testifies to the potential of nanostructure growth for integration of extremely small and low-energy light sources. 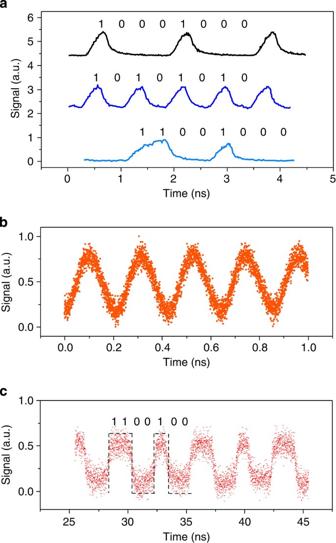Figure 5: Ultrafast nanoresonator device operation. (a) Nanoresonator-based emitters can be directly modulated at 2.5 Gbit s−1. From top to bottom, the traces show light output for modulation patterns 10001000, 10101010 and 11001000, respectively. (b) Meanwhile, devices used as photodetectors can demonstrate clear large signal responses up to 4.6 GHz when averaged. (c) Without averaging, APDs have detected 1 Gbit s−1signals (bit pattern ‘1100100’) with aQfactor of 2.8, demonstrating potential for receiving data real-time. Figure 5: Ultrafast nanoresonator device operation. ( a ) Nanoresonator-based emitters can be directly modulated at 2.5 Gbit s −1 . From top to bottom, the traces show light output for modulation patterns 10001000, 10101010 and 11001000, respectively. ( b ) Meanwhile, devices used as photodetectors can demonstrate clear large signal responses up to 4.6 GHz when averaged. ( c ) Without averaging, APDs have detected 1 Gbit s −1 signals (bit pattern ‘1100100’) with a Q factor of 2.8, demonstrating potential for receiving data real-time. Full size image The APDs developed in this work can operate at similarly high frequencies. Figure 5b shows an averaged large signal response clearly reproducing a 4.6 GHz on-off data stream. Meanwhile, Fig. 5c plots the unaveraged response to a 1-Gbit s −1 pattern of 1100100, showcasing the device’s capacity for real-time high-speed data transport. This particular APD exhibits a Q factor of 2.8, which is modest yet respectable for a first-generation prototype of its kind. Poor light coupling currently limits signal-to-noise performance. Gigahertz operation of both emitters and detectors in this work is rather unprecedented. Prior art with nanowire optoelectronics and other similar nanostructures fails to show ac performance of any sort. Our devices’ gigahertz bandwidths meanwhile fall just short of some of the best commercial devices. This is a major step towards validating as-grown nanostructures as an approach to not only small and exotic but also high-performance photonics. PV power supply Among their many applications, optoelectronics have recently garnered much attention because of their propensity for PV functions. Chip-based nano-optoelectronics are not well suited for solar generation, which demands large-area PV materials. However, exciting examples of non-solar PV applications are emerging, ranging from retinal prosthesis [39] to optical power transfer [40] . In particular, we argue that nanostructure-based PV devices are far better suited as optoelectronic power supplies than solar cells. PV experiments involved devices like the one shown in Fig. 3b , but they were operated in PV mode rather than under reverse bias. 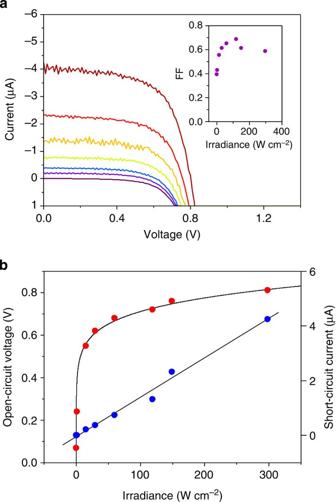Figure 6: PV power supply. (a) Prominent PV effects can be observed from devices under illumination. Going upwards,I–Vcurves correspond to the following irradiance levels: 0, 14.9, 29.8, 59.6, 119, 149 and 298 W cm−2. The inset plots fill factor versus irradiance, which peaks at 0.69. (b) Like many planar III–V junctions,VocandIscincrease versus irradiance in logarithmic and linear fashions, respectively. Under high concentrations,Vocapproaches 0.8 V. Owing to their form factor, nanoscale PV devices are perhaps best suited as power supplies under monochromatic illumination and not as solar cells. Figure 6a plots one particular device’s I – V characteristic under various illumination levels by a 633-nm CW laser, clearly demonstrating power generation. Monochromatic illumination was chosen to simplify experiments and allow us to probe device limits, because solar illumination is an unlikely use case for single nano-optoelectronic devices. As shown in Supplementary Fig. 1 , the ideality factor n can approach 2, a relatively low value for nanostructures, testifying to the quality of our preliminary p–i–n junction design. This is important given the close relationship between ideality factor and PV performance, and future work will focus on reducing n to 1. In Fig. 6b , we find that radial nanopillar junctions [41] behave in a manner similar to most planar junctions. That is, the open-circuit voltage follows a logarithmic dependence on irradiance, while the short-circuit current scales linearly. We can fit the open-circuit voltage curve well using an ideality factor of n =2.3 and a ‘one-sun’ (0.1 W cm −2 ) open-circuit voltage of V oc =0.23 V. Figure 6: PV power supply. ( a ) Prominent PV effects can be observed from devices under illumination. Going upwards, I – V curves correspond to the following irradiance levels: 0, 14.9, 29.8, 59.6, 119, 149 and 298 W cm −2 . The inset plots fill factor versus irradiance, which peaks at 0.69. ( b ) Like many planar III–V junctions, V oc and I sc increase versus irradiance in logarithmic and linear fashions, respectively. Under high concentrations, V oc approaches 0.8 V. Owing to their form factor, nanoscale PV devices are perhaps best suited as power supplies under monochromatic illumination and not as solar cells. Full size image Another figure of merit for PV is fill factor, which is plotted versus irradiance in the inset of Fig. 6a . The fill factor is ~\n0.4 at low irradiance and gradually rises up to 0.69 before settling at ~\n0.6 under very-high laser powers. Meanwhile, the efficiency for a single nanopillar PV device peaks at 51% under high irradiance, approaching the theoretical limit of 58% for 1.96-eV illumination of a 1.13-eV band gap material. This somewhat surprisingly high efficiency may be related to an apparent anomaly. Rigorous calculations ( Supplementary Fig. 6 ) suggest that devices show apparent external quantum efficiency (EQE) exceeding 1. There are indications that this may be due to the natural light concentration properties of nanostructures [27] , [42] , [43] , [44] , [45] , which remains a topic of future investigation. We detail the calculations for our PV experiments in the Methods section. Such high efficiencies are also made possible by using monochromatic irradiance, which can yield nearly perfect PV conversion under the proper conditions [46] . Another advantage of monochromatic illumination is the ability to focus laser light onto a nanoscale PV device for efficient coupling. For sunlight, coupling into such a device presents a major constraint. For these reasons, it thereby proves compelling that PV at the nanoscale may best serve as power supplies for PICs where their energy source is either an on-chip or external laser. In summary, we have shown a pathway towards extremely dense integration of optoelectronic devices into working photonic circuits. Our results highlight how nanostructure growth can complement the rise of silicon photonics by populating these chips with high-performance and small-footprint active III–V devices. In doing so, extremely complex chip-scale optoelectronic functions will emerge with ramifications for myriad applications such as optical interconnects [3] , light detection and ranging [5] , three-dimensional (3D) displays [47] , retinal prosthesis [39] and more. The vertical nature of the nanoresonators presented here may incidentally also facilitate future 3D integrated circuits [14] . Going forward, challenges remain in optimizing junction design as well as wafer-scale material uniformity for improved performance and consistency. Additionally, achieving site-controlled growth of nanoresonators will enable massive scaling of the nanophotonic links shown. Nanoresonator synthesis Growth of nanoresonators first begins with GaAs-based nanoneedles that form on silicon as shown in Supplementary Fig. 7a,b . N-doped (2 × 10 17 cm −3 ) (111) silicon wafers were cleaned with acetone, methanol and deionized water before deoxidizing in buffered oxide etch. After mechanical roughening, the wafers were loaded into an EMCORE D75 MOCVD reactor for growth using tertiarybutylarsine, triethylgallium and trimethylindium sources. Growth occurred at 400 °C after an initial 3-min annealing step at 600 °C. Nanopillar dimensions scaled linearly with growth time; 60 min yields a nominal core diameter of 600 nm using 12 l min −1 hydrogen carrier gas flow. For 12 and 20% InGaAs, trimethylindium mole fractions were 9.86 × 10 −7 and 1.73 × 10 −6 , respectively, while the triethylgallium mole fraction was held at 1.12 × 10 −5 . GaAs layers were grown with a V/III ratio of 48 by simply turning off the indium source. For doping, diethylzinc and diethyltellurium were used with molar fractions ranging from 1 × 10 −7 to 4 × 10 −7 for nominal doping levels of ~\n10 18 cm −3 in both cases. Nanoneedles grow in a conformal core-shell fashion until vertical growth stops and core-shell growth resumes primarily in the radial direction to form nanopillars as illustrated in Supplementary Fig. 7c,d . This enables us to grow radial p–i–n junctions by controlling the composition and doping of each core-shell layer during growth. By finely controlling doping and composition of core-shell layers during growth, we can create a variety of radial diode designs including double heterostructures particularly useful for emitters. There is great freedom in designing the thicknesses and characteristics of each layer, and we discuss some typical diode designs in the next section. With this nanomaterial, we have a platform for creating nano-optoelectronic devices on silicon in a CMOS-friendly manner as depicted in Supplementary Fig. 7e,f . The form factor and geometry nanopillars make them natural nanoresonator structures. Diode heterojunction design During core-shell growth of nanoresonators, we can carefully control the composition and doping level of each layer simply by adjusting indium flow rates and turning doping sources on and off. As a consequence, we can form p–i–n diode heterojunctions in the radial direction. Supplementary Fig. 8 shows two designs we have commonly employed. The first in Supplementary Fig. 8a features a double heterostructure where an n-doped In 0.12 Ga 0.88 As core and p-doped GaAs outer shell function as the higher band gap barriers. Meanwhile, Supplementary Fig. 8b features a similar junction, but with additional intrinsic barrier layers inserted between the doped material and the intrinsic In 0.2 Ga 0.8 As active region. Such a structure is highly favourable for emitter applications, especially lasers. The additional intrinsic layers reduce optical loss by minimizing overlap between lossy dopants and optical modes confined to the active layer. For nanoresonators on silicon, injected current flows through the radial junction from the p-GaAs shell to the n-InGaAs core before travelling downwards into the n-type silicon substrate on which the core is grown. Device fabrication Fabricating devices from single nanopillars involved several steps to spatially register them for nanofabrication processes ranging from e-beam lithography to metallization. Great effort was particularly spent on minimizing leakage current to improve electrical performance of devices. Variations in the process flow occurred depending on the type of device being fabricated. Nonetheless, the following steps are representative of nanoresonator device processing as a whole. 1 Selecting nanoresonators for device fabrication: local and global alignment markers were fabricated on samples using e-beam lithography, metal deposition and metal lift-off processes. These alignment markers functioned to spatially register the locations of select nanoresonators, which were grown spontaneously on silicon at randomized locations. Using SEM, we can map the positions of nanoresonators with respect to known alignment marker coordinates. 2 Etching away shunt paths: during nanoresonator growth, polycrystalline films form on silicon as a by-product. While they do not impact the quality of nanoresonator diodes, the polycrystalline films do create shunt paths for nanoresonator devices. Removing them effectively maximizes shunt resistance. Thus, both dry and wet etching was performed on samples to remove polycrystalline films. To protect the nanoresonators selected for device fabrication during this etching process, we coated them with SiO 2 etch masks. First, plasma-enhanced chemical vapour deposition (PECVD) was used to conformally coat samples with SiO 2 at 300 °C. We then performed e-beam lithography using a negative e-beam resist to coat select nanoresonators with resist. A carefully timed buffered oxide etch then removed SiO 2 everywhere except around select nanoresonators, resulting in an oxide-based etch mask cladding select nanoresonators. SiCl 4 gas was then used to dry etch away most of the polycrystalline film, while a 1:1:30 H 2 SO 4 :H 2 O 2 :H 2 O wet etchant removed any remaining residue. Buffered oxide etch then stripped off the SiO 2 etch masks and cleaned the sample. 3 Electrical isolation: next, a second PECVD process again conformally coated the sample with SiO 2 . Photoresist was then spun onto the chip and etched back using oxygen plasma, exposing the tops of oxide-coated nanoresonators. We then used buffered oxide etch to remove SiO 2 from the upper regions of nanoresonators, exposing their p-GaAs shells for electrical contacts. The photoresist was then removed, and the remaining oxide on the sample functioned to electrically isolate p- and n-layers of the nanoresonator. 4 Metallization: metallization of nanoresonator devices was the final step of the fabrication process flow. Electron beam lithography was used to pattern device contacts and test pads on samples before e-beam metal deposition and lift-off. For APDs and PV devices, samples were mounted at an angle such that the directional metal deposition coated only one side of nanoresonators. This left an aperture open on the other side for external light coupling in our experiments. For stimulated emission devices, nanoresonators were fully embedded in metal by continuously rotating the sample at an angle during e-beam metal deposition. For APD and PV devices, we deposited a thin layer of Ti for adhesion and Au for electrical contacts. For resonant LEDs, thick (300 nm) layers of either silver or gold encapsulated nanoresonators to form metal-optic cavities around them. For silver-based devices, a thin film of gold was first deposited to create Ohmic contacts before silver encapsulation. Photonic link fabrication To demonstrate how optical links can be constructed from grown nanostructures, we used e-beam lithography to write polymer-based waveguides in a simple, three-step process. Negative-tone resist (ma-N 2410) is first spun onto samples, then exposed and subsequently developed to form strip waveguides that run from one nanoresonator-based device to another. Waveguides were laterally tapered at both ends to improve waveguide coupling efficiency of the devices, but no other optimization was done on the waveguide design as it is tangential to the proof of concept in this paper. We note here that we used e-beam lithography in these experiments because our nanostructures grow at randomized locations. Otherwise, our devices are fully compatible with contact lithography as well as all types of waveguides, whether polymer-based or silicon photonic. Low-temperature electroluminescence For electroluminescence (EL) measurements at low temperatures, stimulated emission samples were operated inside a liquid helium-based cryostat that cooled devices down to 4 K. Using silver paste, samples were first mounted onto a leadless chip carrier, which was subsequently mounted onto the cold finger of the cryostat. Wire bonds created electrical connections between devices and the test pads of the leadless chip carrier, which were electrically connected to the electrical feedthroughs of the cryostat. Using these feedthroughs, we were thus able to deliver both CW as well as pulsed current excitation to devices at cryogenic temperatures. For temperature dependence studies, a heater inside the cryostat was used to elevate the temperature of the sample above 4 K. The EL spectrum was recorded using an InGaAs charge-coupled device connected to a spectrometer. Gain modelling In order to estimate how much material gain was achieved from nanoresonators under electrical injection, we fit EL spectra using well-known equations [48] for material gain g and spontaneous emission r sp , as shown inequations (1, 2, 3, 4). Supplementary Table 1 defines the variables in the equations. Supplementary Fig. 4a shows a fit of experimental stimulated emission data (broken blue line) by the theoretically calculated spontaneous emission curve (solid red line). The calculated spectrum nicely fits the background spontaneous emission in the plotted data, which features several stimulated emission peaks superimposed on it. The free parameters used for fitting were carrier concentration and intraband scattering lifetime, which respectively determine the bandwidth of the spectrum and the steepness of its tails. Supplementary Table 2 summarizes the material parameters that were used for the fit. All values represent typical numbers found in literature for InGaAs materials. Where needed, interpolation was used to estimate parameters specifically for In 0.2 Ga 0.8 As. Upon fitting the EL spectrum and extracting carrier concentration and τ in , we have sufficient information to calculate the expected gain spectrum for the device as shown in Supplementary Fig. 4b . From this curve, we see that a high maximum material gain of 3,530 cm −1 has been achieved. At the wavelength corresponding to the experimental stimulated emission peak seen in Supplementary Fig. 4a , the material gain is ~\n3,400 cm −1 . Achieving such high gain truly testifies to the quality of the nanoresonator material grown. These levels of gain approach the limits of typical GaAs-based systems and therefore suggest that our optical cavity, rather than our material, presents the roadblock to achieving electrically-driven nanoresonator lasers on silicon. By optimizing our laser structure design to improve quality factor and gain-mode overlap, we fully expect to achieve this goal in the future. High-speed testing High-speed APD experiments included large-signal, S 21 , and impulse response measurements. To measure impulse responses of APDs, 100-fs laser pulses ( λ =850 nm) functioning as impulse excitations were coupled into devices via a × 20, 0.4 numerical aperture (NA) objective. High-speed RF probes relayed ultrafast photocurrent responses of photodetectors to a bias tee with its RF arm connected to the input of a digital communications analyser (DCA) for measurement and recording. The DCA was triggered by an electrical sync signal from the fs laser used. The DC arm of the bias tee was meanwhile connected to the output of a parameter analyser, which allowed us to bias APDs during measurements and also conduct basic DC characterization. Large-signal and S 21 experiments used a setup similar to the arrangement described above, but with some variation. In particular, an 850 nm vertical-cavity surface-emitting laser (VCSEL) was used as the excitation source because of the ability to directly modulate it at GHz bandwidths. Via a bias tee, we used a pattern generator and a DC bias source to drive the VCSEL and generate user-defined large-signal bit patterns. For small-signal tests, a network analyser was used instead. In both cases, the VCSEL output was collimated and guided in free space to the same × 20, 0.4 NA objective to deliver optical signals for APD photodetection. For large- and small-signal tests, the pattern generator and network analyser triggered the DCA, respectively. All APDs were biased and tested using a pair of closely spaced test pads to accommodate high-speed RF probes. That is, pads for both p-type and n-type contacts were fabricated next to each other on the topside of samples. While an SiO 2 layer electrically isolated p-type contacts and test pads from the n-type Si substrate, SiO 2 was etched away in select areas to expose bare silicon for n-type pad metallization. In this scheme, current would flow along p-type contact fingers and through nanoresonators’ radial diode junctions before routing down into the silicon substrate where it travels back towards the n-type test pad. This design is likely not optimal for high-speed tests and slows the response of our detectors, though as we discuss in the main text, our current bandwidth limitation is due to apparent diffusion processes in nanoresonator junctions. This is evident from the impulse responses of our photodetectors as shown in Supplementary Fig. 5a . Prominent diffusion tails create a ceiling on the bandwidth of our devices, which would otherwise operate much faster. Nonetheless, potential for 10 GHz operation exists as highlighted by Supplementary Fig. 5b , which shows a device’s impulse response with 35-ps rise time (0.35/ τ r =10 GHz). Photonic link operation Photonic link experiments involved using a pattern generator to drive a nanoresonator LED while using either a parameter analyser or oscilloscope in conjunction with a nanoresonator detector at the receiving end. The parameter analyser and oscilloscope were used for dc and ac measurements, respectively. All link experiments were performed at room temperature, and high-speed probes were used for both emitter and detector. Currently, the measurable bandwidth of the link is limited by RF coupling noise between the two sets of probes because they are too close in proximity during testing. This limits out measurements to below 1 kHz, though the devices individually operate at GHz speeds. PV measurement PV experiments were conducted by focusing 633 nm light from a helium–neon (He–Ne) laser onto devices using a × 100, 0.7 NA objective. The spot size (radius) was experimentally measured to be 0.65 μm. The effects of concentration were studied by characterizing PV device performance versus illumination power. Under concentrated irradiance, the open-circuit voltage and short-circuit current behave in a very typical manner as discussed in the main text. While short-circuit current scales linearly with irradiance, open-circuit voltage follows a logarithmic dependence. Because of this, we can estimate the ‘one-sun’ (0.1 W cm −2 ) open-circuit voltage ( V oc ) of our device by fitting our data using equation (5). Here, n , k , T , X and q are ideality factor, Boltzmann constant, temperature, concentration (as a multiple of 0.1 W cm −2 ), and electron charge, respectively. In our fit, we set ideality factor to its measured value of 2.3 while varying V oc until the fit converged onto experimental data at V oc =0.23 V. The temperature T was assumed to be vary with a 4th root dependence on irradiance ( ∝ X 1/4 ) from 20 to 80 °C to take heating effects into account. PV efficiency calculations In order to calculate the conversion efficiency of our PV devices, we must know how much light couples into the nanoresonator. After all, metal cladding the nanoresonator blocks most incident illumination from being absorbed. Furthermore, nanoresonators are 3D structures so absorption is not as easily estimated as for traditional, planar devices. Thus, we performed rigorous finite-difference time-domain calculations to carefully model our experiments and determine how much light couples into the nanoresonator. Supplementary Fig. 6 shows a 3D plot of the normalized absorption per volume for the device characterized in Fig. 4 of the main text. The nanoresonator portion of the device is outlined is white, showing that light couples into the nanoresonator primarily at its base. Metal surrounding the upper portion of the nanoresonator blocks light from being absorbed in that region. Notably, significant absorption occurs in the Au used for electrical contacts. By integrating the absorption per volume over the volumes corresponding to the metal and nanoresonator regions, we calculate the total absorption by each material as a fraction of the excitation source used for our experiment. We found that ~\n6.15% of illumination is absorbed by the nanoresonator while about 6.25% is absorbed by the metal, which receives the vast majority of the incident light. For this particular simulation, we first measured the beam characteristics of the He–Ne source used in our experiments. We then launched an unpolarized Gaussian beam ( λ =633 nm) with beam propagation parameters matching our experimental characterization of the focused He–Ne light. The amount of light absorbed places an upper limit on the possible amount of photogenerated current. Anomalously, we observe photocurrent exceeding this expected amount. In other words, we find that the EQE of our devices appears to exceed 1. As an example, 100 μW of illumination (298 W cm −2 ) through an objective (with measured coupling efficiency of 0.68) should result in absorption of 4.2 μW by the nanoresonator. Given that the wavelength of light used is 633 nm or ~\n2 eV, the maximum photogenerated current is expected to be 2.1 μA assuming perfect internal quantum efficiency and extraction efficiency. However, we have measured up to 4 μA in photocurrent as shown in Fig. 4b of the main text, indicating an apparent device EQE of 1.9. We suspect that this can be explained by the natural capability of nanostructures to concentrate light [42] , [43] , though this requires further investigation and will be a topic for future work. In other words, there are likely additional unknown absorption mechanisms that result in higher absorption than one might traditionally expect. Fully understanding these additional mechanisms and taking them into account will reconcile the apparent EQE and the actual EQE, which indeed should not exceed 1. How to cite this article : Chen, R. et al. Nanophotonic integrated circuits from nanoresonators grown on silicon. Nat. Commun. 5:4325 doi: 10.1038/ncomms5325 (2014).